Direct visualization of microtubules using a genetic tool to analyse radial progenitor-astrocyte continuum in brain Microtubule cytoskeletal dynamics of cortical progenitors and astroglial cells have critical roles in the emergence of normal functional organization of cerebral cortex and in disease processes such as tumorigenesis. However, tools to efficiently visualize these events are lacking. Here we describe a mouse genetic model to efficiently visualize and analyse radial progenitors, their astroglial progeny, and the microtubule cytoskeleton of these cells in the developing and adult brain. Using this tool, we demonstrate altered microtubule organization and capture dynamics in adenomatous polyposis coli-deficient radial progenitors. Further, using multiphoton microscopy, we show the utility of this tool in real-time imaging of astrocytes in living mouse brain and the short-term stable nature of astrocytes in cerebral cortex. Thus, this model will help explore the dynamics of radial progenitor/astrocyte development or dysfunction and the influence of microtubule functions during these events. Radial glial progenitors give rise to most neurons and guide their appropriate migration and placement in the developing cerebral cortex. During late stages of corticogenesis, as neurogenesis and migration dwindles, remaining radial progenitors transform into astrocytes [1] , [2] . Astrocytes contribute to the emergence and maintenance of mature brain circuitry through their function as modulators of neuronal activity, neurogenesis, and as potential neuronal precursors [3] , [4] , [5] , [6] , [7] , [8] , [9] . Radial progenitor development and astroglial polarity depend on dynamic modulation of microtubule cytoskeleton of these cells [10] , [11] , [12] . Genetic mutations or environmental insults affecting the development of radial progenitors and astrocytes can lead to faulty neuronal and glial organization, thus resulting in gross malformations such as lissencephaly and polymicrogyria, as well as in subtle heterotopias [13] , [14] , [15] . Genetic mutations responsible for many of these cortical malformations directly affect microtubule cytoskeletal organization [12] , [13] . Furthermore, the response of differentiated astrocytes to central nervous system (CNS) injuries, from gliosis to generation of new neurons, can be a limiting factor in functional recovery following CNS trauma [16] . A major hurdle in our ability to study and understand the dynamics of astroglial development and function in cerebral cortex is the lack of reliable tools to image large cohorts of developing astroglial cells and their complex cytoskeleton and morphology in the brain. To overcome this deficit, we generated an astroglial specific bacterial artificial chromosome (BAC) transgenic mouse model in which the microtubule cytoskeleton of radial progenitors and their astrocyte progeny in the brain are labelled with GFP, thus providing a powerful tool to directly visualize and analyse normal and aberrant astroglial development in the brain. Generation and characterization of GLAST-EMTB-GFP mice Here the microtubule binding domain of ensconsin fused to GFP (EMTB-3GFP) [17] , [18] is expressed under the transcriptional control of the glutamate-aspartate transporter (GLAST1) regulatory elements [19] ( Fig. 1 ). EMTB-GFP binds and decorates stable microtubules in cells and its expression under the control of the GLAST1 promoter region enables selective cytoskeletal labelling of radial progenitors and their astrocyte progeny from embryonic day 13 onwards in the developing CNS [20] , [21] , [22] . GFP expression can be visualized in freshly vibratomed embryonic cortices in radial progenitors ( Fig. 2 ). Neuronal progeny of these cells appear not to express GFP. Co-immunolabelling of embryonic cortical sections with anti-GFP and neuron-specific Tuj1 antibodies confirms this ( Supplementary Fig. S1 ). Stable, widespread and specific GFP expression in radial progenitors will facilitate the use of this tool in live imaging radial progenitor functions (that is, as proliferating neural progenitors and guides of neuronal migration). Further, GFP-labelled radial progenitor microtubules can be used to analyse the dynamics of radial progenitor microtubule cytoskeleton during these functions ( Fig. 2b,c ; Supplementary Fig. S2 ). 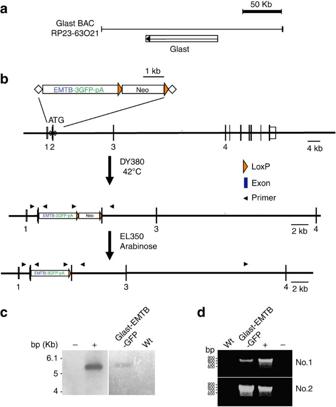Figure 1: Generation of Glast1 promoter-EMTB-GFP mice. (a) Glast1 BAC clone (RP23-63O21), indicating the location of Glast1 gene. (b) Insertion of transgene (EMTB-3GFP-pA) into Glast1 BAC clone. Integration of the transgene by homologous recombination, followed by selection of the targeted BAC clone, and removal of the Neo cassette. Glast1-EMTB-3GFP-pA transgene thus generated was used to drive astroglial specific GFP labelling of stable microtubules in the developing and mature brain. (c) Founder lines were identified by Southern blot analysis of tail DNA and independent breeding lines (namedGlast-EMTB-GFP1,2) were established from two of the founders. (d) PCR products of 808 and 844-bp size were detected with two sets of primers (#1, 2) complementary to 5′ and 3′ arms of Glast-EMTB-GFP DNA. The transgene plasmid was used as a positive control (+ lane) and DNA isolated from wild-type (wt) mice was used as a negative control. Size markers (bp) are indicated in panelscandd. Figure 1: Generation of Glast1 promoter-EMTB-GFP mice. ( a ) Glast1 BAC clone (RP23-63O21), indicating the location of Glast1 gene. ( b ) Insertion of transgene (EMTB-3GFP-pA) into Glast1 BAC clone. Integration of the transgene by homologous recombination, followed by selection of the targeted BAC clone, and removal of the Neo cassette. Glast1-EMTB-3GFP-pA transgene thus generated was used to drive astroglial specific GFP labelling of stable microtubules in the developing and mature brain. ( c ) Founder lines were identified by Southern blot analysis of tail DNA and independent breeding lines (named Glast-EMTB-GFP 1,2 ) were established from two of the founders. ( d ) PCR products of 808 and 844-bp size were detected with two sets of primers (#1, 2) complementary to 5′ and 3′ arms of Glast-EMTB-GFP DNA. The transgene plasmid was used as a positive control (+ lane) and DNA isolated from wild-type (wt) mice was used as a negative control. Size markers (bp) are indicated in panels c and d . 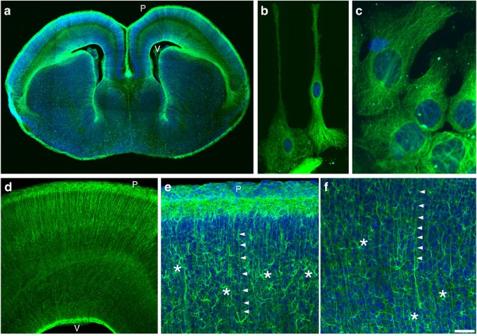Figure 2: Selective labelling of radial progenitors in Glast-EMTB-GFP mice. (a) Prominent labelling of radial progenitors is evident in coronal section from E16 cerebral cortex. (b, c) Microtubule cytoskeleton is clearly labelled in isolated radial progenitors from E16 cerebral cortex. (d) Higher magnification image from E16 dorsal cortex illustrates labelled radial glial scaffold. (e, f) Postnatally, as radial glia transform into astrocytes, both radial processes (arrowheads) and newly formed astrocytes (asterisks) are labelled in P10 cerebral cortex. P, pial surface; V, ventricular surface. Scale bar,a, 300 μm;b, 20 μm;c, 7 μm;d, 75 μm;e,f, 175 μm. Full size image Figure 2: Selective labelling of radial progenitors in Glast-EMTB-GFP mice. ( a ) Prominent labelling of radial progenitors is evident in coronal section from E16 cerebral cortex. ( b, c ) Microtubule cytoskeleton is clearly labelled in isolated radial progenitors from E16 cerebral cortex. ( d ) Higher magnification image from E16 dorsal cortex illustrates labelled radial glial scaffold. ( e, f ) Postnatally, as radial glia transform into astrocytes, both radial processes (arrowheads) and newly formed astrocytes (asterisks) are labelled in P10 cerebral cortex. P, pial surface; V, ventricular surface. Scale bar, a , 300 μm; b , 20 μm; c , 7 μm; d , 75 μm; e , f , 175 μm. Full size image Postnatally, the entire population of astrocytes in the cerebral cortex was labelled very prominently. The complex morphology of astrocytes and the microtubule cytoskeletal underpinnings of this morphology could be clearly visualized ( Figs 2e,f and 3 ). The neurogenic astroglial cells in hippocampal dentate gyrus, anterior subventricular zone and Bergman glia in cerebellum were also labelled ( Fig. 3 ). 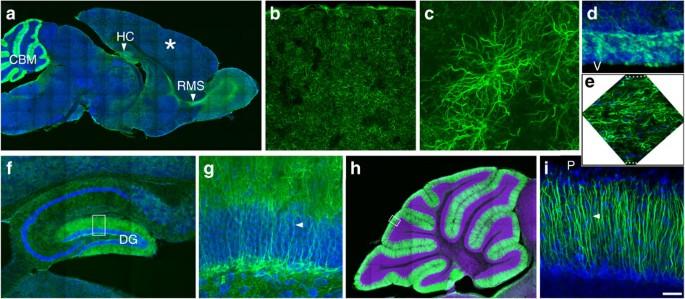Figure 3: Labelling of astrocytes in distinct compartments of the adult brain. (a) A sagittal section from adult Glast-EMTB-GFP brain shows widespread astrocyte labelling in cortical parenchyma (asterisk), hippocampus (HC), rostral migratory stream (RMS), and cerebellum (CBM). (b) Higher magnification view of labelled astrocytes in cortical parenchyma. (c) Imaging of individual cortical astrocytes illustrates the labelling of the astrocyte process network. (d) Labelled astroglial progenitors in the anterior subventricular zone and (e) astrocytes in the rostral migratory stream. (f) In hippocampus, prominent labelling of radial progenitors in dentate gyrus (DG) region, where neurogenesis occurs, is evident. (g) Higher magnification view of outlined area in panel F. Arrowhead indicates radial processes of progenitors. (h) Labelled Bergmann glial cells in cerebellum. (i) Higher magnification view of outlined area in panel H. Arrowhead indicates radial processes of cerebellar Bergmann glial cells. P, pial surface; V, ventricle. Dotted lines in panel E outlines the top and bottom edges of the rostral migratory stream. Scale bar,a, 800 μm;b, 480 μm;c, 52 μm;d,e, 120 μm;f, 330 μm;g, 60 μm;h, 600 μm;i, 50 μm. Figure 3: Labelling of astrocytes in distinct compartments of the adult brain. ( a ) A sagittal section from adult Glast-EMTB-GFP brain shows widespread astrocyte labelling in cortical parenchyma (asterisk), hippocampus (HC), rostral migratory stream (RMS), and cerebellum (CBM). ( b ) Higher magnification view of labelled astrocytes in cortical parenchyma. ( c ) Imaging of individual cortical astrocytes illustrates the labelling of the astrocyte process network. ( d ) Labelled astroglial progenitors in the anterior subventricular zone and ( e ) astrocytes in the rostral migratory stream. ( f ) In hippocampus, prominent labelling of radial progenitors in dentate gyrus (DG) region, where neurogenesis occurs, is evident. ( g ) Higher magnification view of outlined area in panel F. Arrowhead indicates radial processes of progenitors. ( h ) Labelled Bergmann glial cells in cerebellum. ( i ) Higher magnification view of outlined area in panel H. Arrowhead indicates radial processes of cerebellar Bergmann glial cells. P, pial surface; V, ventricle. Dotted lines in panel E outlines the top and bottom edges of the rostral migratory stream. Scale bar, a , 800 μm; b , 480 μm; c , 52 μm; d , e , 120 μm; f , 330 μm; g , 60 μm; h , 600 μm; i , 50 μm. Full size image Viability and fertility of these mice were identical to that of wild-type mice. Gross examination of brains and other organs such as heart, lungs, liver and kidney of these mice did not indicate any changes ( Supplementary Table S1 ). Further, Ensconsin microtubule domain binds to stable microtubules without affecting microtubule dynamics. Post-translational modifications such as acetylation or detyrosination distinguish the stable forms of microtubules [23] . Evaluation of the levels of acetylated tubulin (aged, stable form of tubulin) or detyrosinated tubulin (post-translationally modified stable microtubules) in Glast-EMTB-GFP mice indicates no significant changes in the levels of stable microtubules ( Supplementary Fig. S3 ), thus confirming that EMTB-GFP labelling does not affect microtubule stability in these mice. Further, in vitro , GFP expression levels did not differ significantly between cells maintained in defined medium (Neurobasal/N2/B27) or serum-supplemented medium (DMEM/10% fetal bovine serum). The average GFP fluorescent intensity (a.u.) of cells maintained in NB/N2/B27 and DMEM/FBS were 5.7±0.56 ( n =20) and 5.4±0.49 ( n =20), respectively. Live imaging of astroglial cells in Glast-EMTB-GFP mice To determine the use of this tool for live imaging of astroglial cells in vivo , we directly visualized astroglial cells in living mice using multiphoton microscopy ( Fig. 4a,b ). Imaging was carried out through a circular cranial window. Both open and thin skull windows were used for in vivo imaging. GFP-labelled astrocytes and their association with blood vessels were imaged several hundred micrometers deep in the cerebral cortex of living mice. To examine the dynamics of cortical astroglial cells in vivo , we repeatedly imaged same cortical astroglial cell processes at 20-min intervals in living mice. Astroglial processes that are intercalated between cortical neurons in vivo were stable and do not undergo rapid short-term changes ( Fig. 4c,d ). Further, dynamics of the microtubule cytoskeleton in astroglial cells can be easily visualized. Changing dynamics of the microtubule cytoskeleton in migrating astroglial cells, in astroglial cells in contact with other astroglia, individual microtubule filament extension, retraction or branching, and organizational changes of the microtubule cage around nuclei can be imaged in real time ( Fig. 5 ; Supplementary Fig. S3 ; Supplementary Movies 1 , 2 , 3 , 4 and 5 ). 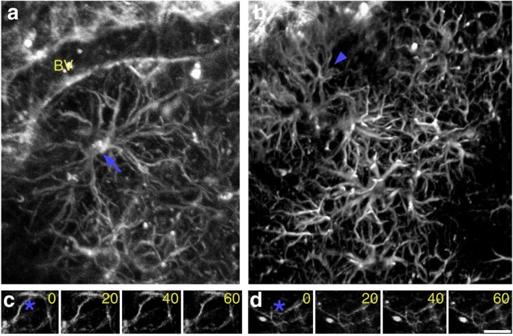Figure 4:In vivomultiphoton microscopy of labelled astrocytes in living adult Glast-EMTB-GFP mice. Labelled astrocytes in somatosensory region of cerebral cortex were imaged through a cranial window at a depth of 250 μm (a) or 350 μm (b) from the pial surface. The complex morphology of astrocytes (arrow,a), their corresponding processes (arrowhead,b), and the astrocytic end-feet contacts with the blood vessels (BV,a) can be distinguished. (c,d) Time lapse imaging of astroglial processesin vivoindicates that these processes are stable over the short term (compare processes adjacent to asterisks). Time elapsed between frames are indicated in minutes. Scale bar, 27 μm. Figure 4: In vivo multiphoton microscopy of labelled astrocytes in living adult Glast-EMTB-GFP mice. Labelled astrocytes in somatosensory region of cerebral cortex were imaged through a cranial window at a depth of 250 μm ( a ) or 350 μm ( b ) from the pial surface. The complex morphology of astrocytes (arrow, a ), their corresponding processes (arrowhead, b ), and the astrocytic end-feet contacts with the blood vessels (BV, a ) can be distinguished. ( c , d ) Time lapse imaging of astroglial processes in vivo indicates that these processes are stable over the short term (compare processes adjacent to asterisks). Time elapsed between frames are indicated in minutes. Scale bar, 27 μm. 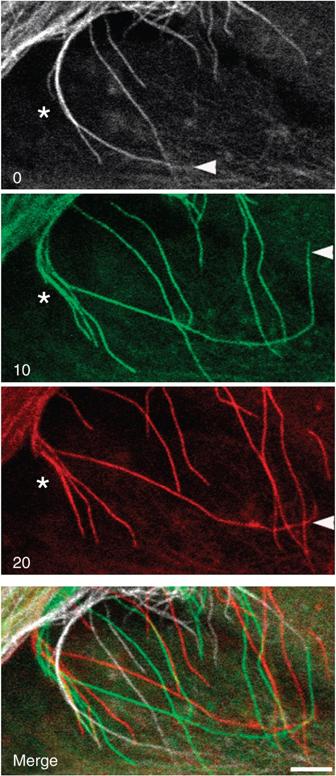Figure 5: Dynamics of microtubule filaments. Growth, shortening or branching of individual microtubule filaments can be seen in this time-lapse panel (see filaments adjacent to arrowhead (growth and shortening) or asterisk (branching)). Merged panel shows the extent of rearrangements over time. Panels were taken from a section ofSupplementary Movie 4(from 1.00 to 1.20 time frames). Time elapsed between frames are indicated in minutes. Scale bar, 5 μm. Full size image Figure 5: Dynamics of microtubule filaments. Growth, shortening or branching of individual microtubule filaments can be seen in this time-lapse panel (see filaments adjacent to arrowhead (growth and shortening) or asterisk (branching)). Merged panel shows the extent of rearrangements over time. Panels were taken from a section of Supplementary Movie 4 (from 1.00 to 1.20 time frames). Time elapsed between frames are indicated in minutes. Scale bar, 5 μm. Full size image Altered microtubule dynamics in APC deficient radial progenitors To examine the utility of these mice in deciphering microtubule dynamics underlying radial progenitor functions, we generated conditional mutants of APC in which APC-deficient radial progenitors express EMTB-GFP. APC serves an essential function in the maintenance of polarized radial glial scaffold during brain development [10] . APC was inactivated in the radial progenitors of embryonic cerebral cortex using an APC-floxed allele line (APC Lox/Lox ) and the hGFAP promoter-Cre line that drives Cre recombinase in developing radial progenitors [10] . To visualize microtubules in APC deficient radial progenitors, we generated hGFAP-Cre; APC Lox/Lox ; Glast-EMTB-GFP mice. Littermate hGFAP-Cre; APC Lox/+ ; Glast-EMTB-GFP mice were used as controls. Live imaging of radial progenitors from these mice (E16) indicates that, compared with controls, microtubules in APC-deficient radial progenitors are highly disorganized. At the tips of radial progenitors, APC deficient microtubules appear not to be able to extend, branch and retract as in controls, instead, they tend to swirl and form loops in an unorganized manner ( Supplementary Movies 6 , 7 , 8 ). Increased numbers of microtubules with kinked, hairpin loop-like organization was seen in the cortical region of APC-deficient cells ( Fig. 6 ; Supplementary Movie 8 ). They may represent microtubules that were unable to undergo cortical capture and anchoring at the cell membrane in the absence of APC, as APC is thought to be part of the complex critical for microtubule capture. APC-regulated microtubule capture at the cell cortex is considered to be essential to maintain cell polarity and for targeted delivery of signalling molecules involved in cell–cell interactions [24] , [25] , [26] . Further, in the radial process of APC-deficient radial progenitors, an increase in microtubule disorganization preceded the collapse of these processes ( Supplementary Movies 9 , 10 and 11 ). These observations validate the use of Glast-EMTB-GFP mice in revealing a hitherto undefined aspect of microtubule disorganization resulting from APC deletion in radial progenitors and how this may contribute to the APC regulated morphological polarity of radial progenitors in the cerebral cortex. 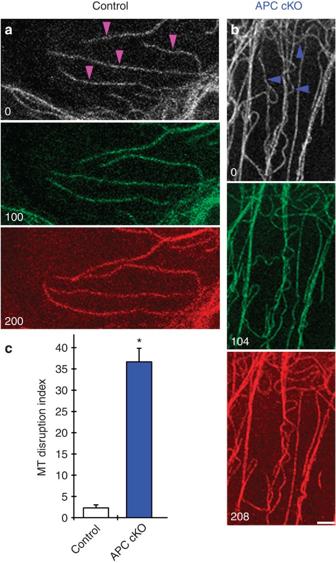Figure 6: Disrupted microtubule organization in APC-deficient radial progenitors. Labelled microtubule filaments in cortical regions of control (hGFAP-Cre; APCLox/+; Glast-EMTB-GFP) and APC deficient (hGFAP-Cre; APCLox/Lox; Glast-EMTB-GFP [APC cKO]) radial progenitors were repeatedly imaged. Growth, shortening and branching of individual microtubule filaments (arrowheads,a) can be seen in control cells. In contrast, significant numbers of APC-deficient microtubule filaments are kinked and appear to have hairpin loop-like shape (arrowheads,b). (c) Quantification of kinked, hairpin loop-like microtubule filaments in control (n=66) and APC cKO (n=37) radial progenitors indicates a significant increase in APC cKO cells. Percentages of hairpin loop-like microtubule filaments in 150 μm2cortical area were measured and used as microtubule (MT) disruption index. Time elapsed between frames are indicated in seconds. Data shown are mean±s.e.m.; asterisk, significant when compared with controls atP<0.01 (Student'sttest). Scale bar, 2.5 μm. Also seeSupplementary Movie 9. Figure 6: Disrupted microtubule organization in APC-deficient radial progenitors. Labelled microtubule filaments in cortical regions of control (hGFAP-Cre; APC Lox/+ ; Glast-EMTB-GFP) and APC deficient (hGFAP-Cre; APC Lox/Lox ; Glast-EMTB-GFP [APC cKO]) radial progenitors were repeatedly imaged. Growth, shortening and branching of individual microtubule filaments (arrowheads, a ) can be seen in control cells. In contrast, significant numbers of APC-deficient microtubule filaments are kinked and appear to have hairpin loop-like shape (arrowheads, b ). ( c ) Quantification of kinked, hairpin loop-like microtubule filaments in control ( n =66) and APC cKO ( n =37) radial progenitors indicates a significant increase in APC cKO cells. Percentages of hairpin loop-like microtubule filaments in 150 μm 2 cortical area were measured and used as microtubule (MT) disruption index. Time elapsed between frames are indicated in seconds. Data shown are mean±s.e.m. ; asterisk, significant when compared with controls at P <0.01 (Student's t test). Scale bar, 2.5 μm. Also see Supplementary Movie 9 . Full size image This approach of inertly tagging the microtubule cytoskeleton in a cell-type-specific (that is, radial progenitor-astroglial) manner in the CNS provides several advantages. First, GFP labelling of stable microtubules in these cells enables clear and unambiguous visualization of the morphology and dynamics of these cells in vitro and in vivo . Weak GFP expression in the cytoplasm of previously established astroglial indicator mice precludes such visualization in living tissue [16] . Widespread and stable labelling of astroglial cells of the cerebral cortex, hippocampus, midbrain and cerebellum highlights the utility of these mice as a tool for the analysis of the radial progenitor–astrocyte continuum in distinct compartments of the developing and adult mammalian brain. It will help evaluate the contributions of these cells to neurogenesis, guidance of neuronal migration, and formation and maintenance of neuronal synaptic connections. Long-term co-imaging of astroglia and adjacent neuronal dendritic spines in these mice may help examine the reciprocal influences astroglia exert on cortical neuronal microcircuit dynamics. Second, the microtubule cytoskeleton is critical for proliferation, polarization, and morphological organization of radial progenitors and astroglia. Our transgenic approach labels radial glial and astrocyte microtubules without interfering with their normal function. Microtubules in these cells can be visualized immediately without the need for any cumbersome procedures to label microtubules before imaging. Thus, as shown with APC mutants, it will serve as an efficient tool in exploring the dynamics of microtubule functions during radial progenitor/astrocyte development or dysfunction. Finally, when crossed with mouse mutant models of astroglioma or neurodevelopmental disorders with astroglial dysfunctions, these mice will help us evaluate how astroglial dysfunction may underlie tumorigensis or the pathogenesis of neurodevelopmental disorders such as epilepsy, schizophrenia and autism. Construction of GLAST1-EMTB-GFP BAC transgene construct EMTB-3XGFP-pA (gift from Dr J.C. Bulinski, Columbia University) was cloned into pBlueScript KSII (Stratagene). A FRT em7-Neo cassette was then inserted at MfeI site before SV40 polyA signal to introduce Neo as a selection marker for recombineering and to provide extra unique sites of restriction endonuclease to ligate with homologous arms for targeting. Using overlapping PCR, restriction enzyme sites, Nde I and Pme I, were added in between homologous arms. EMTB-3XGFP-FRT-Neo was then inserted into the Pme I site. After excising targeting cassette and performing BAC targeting, EMTB-3XGFP-FRT-Neo was inserted into GLAST exon 2 (ATG exon) within C57 mouse BAC [RP23-63O21], replacing the exon 2 sequence (−8 ∼ +5), including the initiation codon ( Fig. 1 ). Neo cassette in the targeted GLAST BAC was deleted by Flpe induction in EL 250 bacteria. Generation of BAC transgenic mice Purified BAC was used for pronuclear microinjection of fertilized eggs from the CBA X C57Bl6 mouse strain at the UNC animal model core facility. Fertilized ova were subsequently implanted into pseudo-pregnant females and offspring were analysed for the insertion of the BAC construct. Founder lines were identified by Southern blot analysis of tail DNA ( Fig. 1c ). An [α- 32 P] dCTP-labelled DNA probe was generated from a 1337 bp NheI-BsrGI fragment of the EMTB-GFP region of the BAC construct and used to probe the DNA blot. Independent breeding lines were established from two of the founders (named Glast-EMTB-GFP 1,2 ) and subsequent offspring were analysed by PCR, using the following two primer sets, 5′-CCA ACC CTG AAG AAC CCC TTA C-3′ and 5′-TCT GGC TCC TTT CCA TTG TGC 3′-(No. 1); 5′-AAA AAA CCT CCC ACA CCT CCC C-3′ and 5′-ATA ACA CCC CCC AGG CAT TCA TGC-3′ (No. 2) complementary to 5′ and 3′ arms of the GLAST1-EMTB-GFP transgene, respectively. Both founder lines expressed identical patterns of GFP expression. Glast-EMTB-GFP lines were maintained on a C57Bl6 background and all animals were housed under identical conditions. These mice were normal and fertile ( Supplementary Table 1 ). Heterozygous mice were used in these studies. All procedures were carried out in accordance with NIH guidelines and the University of North Carolina's animal care and use committee guidelines. hGFAP-Cre; APC lox / lox ; Glast-EMTB-GFP Mice Radial progenitor-specific conditional knockout APC mice (APC lox/lox ; hGFAP-Cre) were generated by mating mice carrying an APC allele flanked by lox P sites with hGFAP-Cre mice [10] . Progeny from APC lox/+ ; hGFAP-Cre + and Glast-EMTB-GFP matings were used to generate APC lox/lox ; hGFAP-Cre; Glast-EMTB-GFP mice. Radial progenitors from these mice were then isolated and imaged [10] . Immunohistochemistry Immunohistochemical labelling of embryonic and postnatal brain sections or isolated astroglial cell was performed, as described earlier [10] . The following primary antibodies were used: RC2 (undiluted supernatant; Iowa Hybridoma Bank), anti-BLBP (1:500; Chemicon), anti-GFAP (1:500; Sigma), anti-GFP (1:1000; Abcam), and Tuj-1 (1:500; Chemicon). Appropriate Cy2, Cy3, or Alexa dye conjugated secondary antibodies (Jackson ImmunoResearch, Molecular Probes) were used to detect primary antibody binding. DRAQ5 (Alexis) or Hoechst 33258 (Molecular probes) was used as nuclear counterstain. In vivo two-photon laser scanning microscopy of astroglial cells Postnatal (P30) mice were anesthetized using avertin (0.2 ml per 10 g body weight) and an ∼ 1 mm opening in the skull was made above somatosensory cortical region as described earlier [27] . In some experiments, a thinned-skull cranial window was created instead [28] . An optical stage containing the immobilized mouse was attached to a Zeiss LSM710 multiphoton microscope, and in vivo images of GFP expressing astroglial cells in a depth of 250–350μm were acquired using a X20 objective. Live imaging of microtubule dynamics in astroglial cells Astroglial cells from postnatal day-7 SVZ were cultured as described in Anton et al . [29] Nuclei were labelled with Hoechst 33258. GFP + microtubules in these cells were repeatedly imaged at 5–10 min intervals using a ×63 objective in an Olympus FV1000 confocal microscope equipped with live-cell incubation chamber. The background normalized GFP fluorescence intensities (arbitrary units (a.u.)) of astroglial cells maintained in Neurobasal/N2/B27, or DMEM/10%FBS were measured using Zeiss LSM image browser and Image J program. How to cite this article: Eom, T.-Y. et al . Direct visualization of microtubules using a genetic tool to analyse radial progenitor-astrocyte continuum in mice. Nat. Commun. 2:446 doi: 10.1038/ncomms1460 (2011).